Environmental fatty acids enable emergence of infectiousStaphylococcus aureusresistant to FASII-targeted antimicrobials The bacterial pathway for fatty acid biosynthesis, FASII, is a target for development of new anti-staphylococcal drugs. This strategy is based on previous reports indicating that self-synthesized fatty acids appear to be indispensable for Staphylococcus aureus growth and virulence, although other bacteria can use exogenous fatty acids to compensate FASII inhibition. Here we report that staphylococci can become resistant to the FASII-targeted inhibitor triclosan via high frequency mutations in fabD , one of the FASII genes. The fabD mutants can be conditional for FASII and not require exogenous fatty acids for normal growth, and can use diverse fatty acid combinations (including host fatty acids) when FASII is blocked. These mutants show cross-resistance to inhibitors of other FASII enzymes and are infectious in mice. Clinical isolates bearing fabD polymorphisms also bypass FASII inhibition. We propose that fatty acid-rich environments within the host, in the presence of FASII inhibitors, might favour the emergence of staphylococcal strains displaying resistance to multiple FASII inhibitors. S taphylococcus aureus is a remarkably versatile opportunist pathogen that has confounded the medical community by its ability to escape antibiotic inhibition. Multidrug-resistant S. aureus are a main cause of hospital- and community-acquired infections, and treatment constitutes a major medical and economic challenge [1] , [2] . The fatty acid synthesis pathway (FASII) has been a leading candidate as a novel essential target for antimicrobial discovery. Numerous FASII inhibitors are in the pipeline or in clinical trials, most of which target FabI, the enoyl-acyl carrier protein (ACP) reductase (for example, AFN-1252 (now Debio-1452 and pro-drug Debio-1450), CG400549, CG400462 and MUT056399), or FabF, the β-ketoacyl-ACP synthase (for example, platencin, platensimycin and fasamycins A and B) [3] , [4] , [5] , [6] , [7] , [8] , [9] , [10] , [11] . Triclosan, a chemically synthesized biocide first introduced in 1965, is the best known FabI inhibitor developed thus far, and has had widespread use in hygiene, health care, and household products at concentrations of up to 1% (refs 12 , 13 ). In consequence, triclosan detection in human fluids is common, and has generated information on the limits of use of this anti-FASII, including safety issues [14] , [15] , [16] , [17] , [18] , [19] . Observed side effects of triclosan on the host may be caused by its general membrane-disrupting activity [12] , [17] , [19] . Additionally, triclosan-resistant staphylococci, conferred by mutations that maintain FASII activity, or obtained by horizontal transfer of the Staphylococcus haemolyticus fabI gene (encoding a naturally occurring resistant FabI variant), are estimated to comprise 5–15% of S. aureus clinical isolates [14] , [16] , [20] . Continued anti-FASII development is based on development of antimicrobials with greater FabI affinity and specificity that would curb its potentially dangerous side effects [4] , [9] , [21] , [22] , [23] , [24] . However, fatty acids are abundant in the host and can be used by several Gram-positive pathogens to overcome a FASII deficiency [25] , [26] , [27] , [28] , which questions FASII targeting as a general strategy for antibacterial drug discovery. For example, exogenous fatty acids can fully compensate a FASII deficiency in Streptococcus agalactiae , and a FASII auxotroph was fully virulent in a murine septicaemic infection model [25] . Nevertheless, the ability of S. aureus to override FASII inhibition in the presence of fatty acids has remained in question [4] , [21] , [26] , [29] , [30] . S. aureus FASII expression is not blocked by exogenous fatty acids, whereas it is inhibited in streptococci [21] . Rather than synthesizing unsaturated fatty acids to fluidify their membranes (as do the streptococci), S. aureus synthesizes branched chain fatty acids, of which the main one, anteiso C15:0 ( ai 15:0), is apparently required for phospholipid synthesis [27] , [31] , [32] . Moreover, it has been proposed that FASII inhibition in S. aureus leads to accumulation of acyl-ACP intermediates, thereby limiting ACP availability for exogenous fatty acid utilization [9] , [27] , [33] , [34] (see Supplementary Figs 1 and 2 for pathway and genetic contexts). In addition, while fatty acid auxotrophs (defective in acc genes encoding acetyl-CoA carboxylase) are viable, optimal growth requires ai 15:0, and these acc mutants are avirulent in a mouse septicaemic infection model [24] , [27] , [32] . The fundamental and medical importance of FASII-targeted drug development incited us to characterize S. aureus responses to anti-FASII drugs. Here we show that fatty acids, which are ubiquitous host constituents, can facilitate the emergence of S. aureus resistance to anti-FASII drugs. Fatty acids facilitate the emergence of triclosan resistance Some Gram-positive bacteria can incorporate exogenous fatty acids, which enable resistance to anti-FASII drugs [25] , [26] . In the case of S. aureus , we considered the possibility that arising mutations could facilitate fatty acid incorporation and lead to FASII bypass, as hypothesized in an earlier study [27] . To reveal such fatty-acid-based triclosan resistant (FA-T R ) mutants, we examined the response of the S. aureus Newman strain to the FabI inhibitor triclosan on fatty-acid-containing BHI solid medium. A fatty acid cocktail (referred hereafter as ‘FA’) was used comprising C14:0, C16:0, and C18:1, which are present in the human host [35] , [36] . Overnight S. aureus BHI cultures were plated on medium containing FA and 0.25 μg ml −1 triclosan; as controls, they were also plated on medium without FA and/or triclosan. Triclosan-resistant colonies arose at about 100-fold higher frequencies ( ∼ 10 −6 ) in the presence of FA. The FA-T R colonies were screened for growth on BHI, BHI-triclosan (BHI-T), BHI-FA and BHI-FA-triclosan (BHI-FA-T) plates ( Supplementary Fig. 3 ). A minority of clones grew on all four media (FA prototroph triclosan resistant mutants, T R mutants). The remaining clones grew either on BHI, BHI-FA and BHI-FA-T (FA prototrophs), or on FA-containing media but very poorly or not at all on BHI. The latter were thus considered as fatty-acid-dependent for normal growth and were designated DepT R mutants. Fatty acids thus appear to facilitate the emergence of triclosan resistance in S. aureus . Three classes of S. aureus FA-T R mutants Fatty acid profiles of randomly selected FA-T R mutants (16 prototrophs and 20 DepT R mutants) were determined from whole cell extracts of cultures prepared in BHI-FA-T medium. Representative profiles of each class of mutants are shown ( Fig. 1 ). Among prototrophs, a minor class (3/16) comprised mutants with endogenous (EndoT R ) fatty acid profiles, indicating that the FASII pathway was active. The dominant class of prototrophs (13/16) comprised mutants having media-dependent fatty acid profiles, that is, with exogenous fatty acids in BHI-FA-T, and endogenous fatty acids in BHI (conditional triclosan-resistant mutants, referred to as CondT R ). Mutants of this class have not previously been reported. All the DepT R clones showed poor or no growth on BHI plates, but displayed exogenous profiles in BHI-FA-T medium. These results show that the majority of isolated FA-T R mutants were able to bypass a FASII block by incorporating exogenous fatty acids. 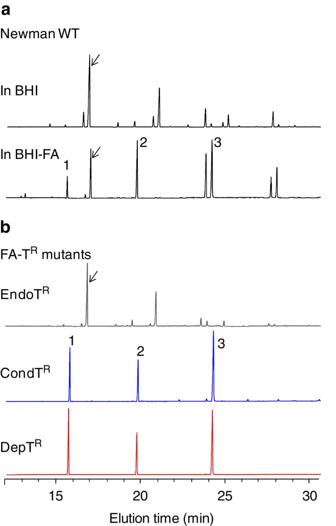Figure 1:S. aureusNewman WT and FA-TRmutants use exogenous fatty acids. Fatty acid profiles are shown for (a) Newman strain (WT) cultures grown in BHI and BHI-FA and (b) FA-TRclones grown in BHI-FA-T.S. aureussynthesizes branched chain fatty acidsde novo, mainly C15:0 (ai15:0; indicated by arrow) and its elongation products, and saturated straight chain fatty acids. In BHI-FA, the WT strain uses exogenous fatty acids, but continuesde novosynthesis. Peaks 1, 2, and 3 correspond to the exogenous fatty acids added during growth, respectively C14:0, C16:0, and C18:1 (collectively referred to as ‘FA’, see Methods). EndoTR, FA-TRwith endogenous fatty acids (grey); CondTR, FA-TRwith conditional FASII activity (blue), that is, active in BHI but bypassed in fatty acids plus triclosan; DepTR, FA-TRrequiring exogenous fatty acids for growth (red). The fatty acid profile of the EndoTRmutant was similar to that of the WT in BHI, while CondTRand DepTRprofiles are exogenous. Figure 1: S. aureus Newman WT and FA-T R mutants use exogenous fatty acids. Fatty acid profiles are shown for ( a ) Newman strain (WT) cultures grown in BHI and BHI-FA and ( b ) FA-T R clones grown in BHI-FA-T. S. aureus synthesizes branched chain fatty acids de novo , mainly C15:0 ( ai 15:0; indicated by arrow) and its elongation products, and saturated straight chain fatty acids. In BHI-FA, the WT strain uses exogenous fatty acids, but continues de novo synthesis. Peaks 1, 2, and 3 correspond to the exogenous fatty acids added during growth, respectively C14:0, C16:0, and C18:1 (collectively referred to as ‘FA’, see Methods). EndoT R , FA-T R with endogenous fatty acids (grey); CondT R , FA-T R with conditional FASII activity (blue), that is, active in BHI but bypassed in fatty acids plus triclosan; DepT R , FA-T R requiring exogenous fatty acids for growth (red). The fatty acid profile of the EndoT R mutant was similar to that of the WT in BHI, while CondT R and DepT R profiles are exogenous. Full size image Gain of function in an S. aureus conditional mutant Growth and fatty acid profiles of CondT R -17 and the Newman strain were compared in the absence or presence of fatty acids and triclosan ( Fig. 2a ). Growth of both strains was comparable in BHI medium. The addition of fatty acids expectedly slowed strain growth, which was also comparable for both strains ( Fig. 2a , centre) [37] , [38] . When triclosan was added, CondT R -17 maintained growth, but not the Newman strain. Fatty acid profiles confirmed CondT R strain capacity to bypass FASII inhibition and shift to the exogenous FA source ( Fig. 2b ). Thus, this conditional mutant can use exogenous fatty acids upon FASII block, while displaying normal growth otherwise. 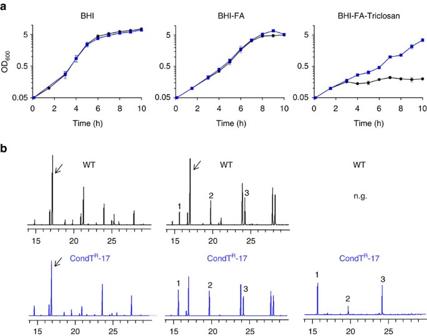Figure 2: Gain of function of theS. aureusCondTR-17 mutant. (a) Growth of WT and CondTR-17 (fabDG196R)S. aureusstrains in BHI, BHI-FA and BHI-FA-T media. Results show the average and range of biologically independent duplicates. (b) Fatty acid profiles of one sample set, taken at the 10 h time point. Endogenous branched-chain fatty acid (ai15:0) is indicated with arrows. Fatty acids are: 1- C14:0; 2- C16:0 and 3- C18:1, the fatty acids comprised in BHI-FA-T medium. N.g., no growth. Black, WT; blue, CondTR-17. Figure 2: Gain of function of the S. aureus CondT R -17 mutant. ( a ) Growth of WT and CondT R -17 ( fabD G196R ) S. aureus strains in BHI, BHI-FA and BHI-FA-T media. Results show the average and range of biologically independent duplicates. ( b ) Fatty acid profiles of one sample set, taken at the 10 h time point. Endogenous branched-chain fatty acid ( ai 15:0) is indicated with arrows. Fatty acids are: 1- C14:0; 2- C16:0 and 3- C18:1, the fatty acids comprised in BHI-FA-T medium. N.g., no growth. Black, WT; blue, CondT R -17. Full size image Numerous FASII-bypass mutations map to fabD Known S. aureus triclosan-resistant mutants carry mutations in the gene encoding FabI, the triclosan target: such mutant enzymes fail to bind triclosan but remain enzymatically active [12] , [14] , [16] , [24] . Our FA-T R clones with EndoT R fatty acid profiles resembled previously described strains carrying mutations in fabI [14] , [16] . The role of fatty acids in obtaining such mutants is unknown. In contrast, all tested mutants with exogenous fatty acid profiles (DepT R and CondT R strains) carried wild type fabI genes ( Table 1 ). Table 1 Characterization of FA-T R mutants. Full size table Previously isolated S. aureus fatty acid auxotrophs mapped to FASII initiation genes accC and accD , encoding acetyl-CoA carboxylase subunits (biotin carboxylase and β-carboxytransferase respectively) for malonyl-CoA synthesis [27] ( Supplementary Fig. 1 ). Among five tested DepT R mutants, one (DepT R -28) carried an accB mutation ( Table 1 ). Whole genome sequencing of one CondT R and three DepT R mutants revealed that these mutants carried fabD mutations as compared with the Newman parental strain ( Table 1 , sequenced strains are designated with ‘#’). CondT R -17 bore a single nucleotide substitution generating FabD G196R ; DepT R -5 carried a single nucleotide insertion that truncated FabD at amino acid position 8. No other mutation was detected in either strain. Strains DepT R -45 and DepT R -72 displayed single nucleotide deletions in fabD , and each carried a second mutated allele ( Table 1 ), which mapped to either NWMN_0043 encoding conserved Staphylococcal Antigen 1b (Csa1b), one of a conserved family of 18 protein homologues [39] (for DepT R -45), or NWMN_1735, encoding a DNA-repair-related protein [40] (for DepT R -72). We chose to focus here on the singly mutated fabD strains. Sequencing fabD of other FA-T R CondT R clones revealed mutations mainly at position G196, and one at position Q265 ( Table 1 ). FabD G196 is adjacent to key residues (positions 198 and 199) of the FabD active site based on S. aureus FabD crystallography [41] ; it is possible that substitution by less flexible amino acids than glycine might impose constraints on FabD activity. The Q265P mutation is within a conserved region separating a helix from a β-strand as suggested from Escherichia coli FabD structure [42] . Thus, the majority of FA-T R S. aureus mutants identified here contain mutations in fabD and utilize exogenous fatty acids to overcome FASII inhibition. Both fabD and acc intervene in FASII initiation ( Supplementary Fig. 1 ), suggesting the importance of this first step in FASII bypass [27] . Diverse fatty acid combinations allow FASII bypass Previous studies suggested that ai 15:0 was strictly required at the second acyl position of the S. aureus phospholipid [24] , [27] , [32] , [43] . However, our results indicated that other fatty acids can replace ai 15:0. We explored the possibility that a fatty acid of similar length, like C14:0 (33% of our FA cocktail), might substitute for ai 15:0 when FASII was blocked ( Fig. 3 ). The DepT R -5 mutant was grown in medium containing triclosan and fatty acid cocktails with 33, 3 or 0% C14:0. For each cocktail, the amounts of C14:0 in S. aureus profiles reflected its proportions among fatty acids in the medium, indicating that C14:0 is not preferentially incorporated for FASII bypass. 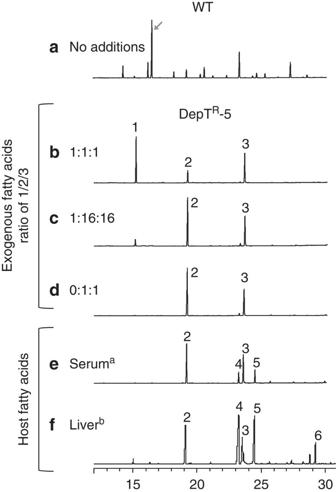Figure 3: AS. aureus fabDmutant uses diverse fatty acid combinations for FASII bypass. (a) Newman strain in BHI. (b–f) Cultures of DepTR-5 were grown in BHI medium supplemented with triclosan and different fatty acid combinations and ratios, as indicated. Fatty acid profiles and OD600were determined on cells harvested from 7.5 h (a–e) and 4.5 h (f) cultures.a, medium was supplemented with 10% delipidated serum, which lowered toxicity.b, Liver extract, prepared by sterile filtration, was added at a final concentration of 3% (without added fatty acids). The diagonal arrow indicates the position ofai15:0, the major fatty acid synthesized byS. aureus. Fatty acids are: 1- C14:0; 2- C16:0; 3- C18:1; 4- C18:0; 5- C18:2; 6- C20:4. Proportions of input fatty acids present in supplemented media are indicated at left. Fatty acid profile of liver extract is inSupplementary Fig. 4. Figure 3: A S. aureus fabD mutant uses diverse fatty acid combinations for FASII bypass. ( a ) Newman strain in BHI. ( b – f ) Cultures of DepT R -5 were grown in BHI medium supplemented with triclosan and different fatty acid combinations and ratios, as indicated. Fatty acid profiles and OD 600 were determined on cells harvested from 7.5 h ( a – e ) and 4.5 h ( f ) cultures. a , medium was supplemented with 10% delipidated serum, which lowered toxicity. b , Liver extract, prepared by sterile filtration, was added at a final concentration of 3% (without added fatty acids). The diagonal arrow indicates the position of ai 15:0, the major fatty acid synthesized by S. aureus . Fatty acids are: 1- C14:0; 2- C16:0; 3- C18:1; 4- C18:0; 5- C18:2; 6- C20:4. Proportions of input fatty acids present in supplemented media are indicated at left. Fatty acid profile of liver extract is in Supplementary Fig. 4 . Full size image A mix of the four principal fatty acids in human serum in physiological proportions (C16:0, C18:0, C18:1 and C18:2) was also tested. When added in purified form, the free fatty acid cocktail was toxic to staphylococci, likely due to C18:2 (linoleic acid), which makes up ∼ 35% of serum fatty acids [35] . However, growth was restored when 10% delipidated serum was added, and DepT R -5 displayed an exogenous fatty acid profile ( Fig. 3e ). To mimic the within-host environment during infection, we grew S. aureus wild type and DepT R -5 strains in medium containing sterile-filtered pig liver and kidney extracts. The incorporated fatty acids reflected those present in the medium (shown for liver; Fig. 3f , see Supplementary Fig. 4 for organ extract profile). Unexpectedly, long-chain unsaturated fatty acids C18:2 and C20:4 were efficiently incorporated. C16:0 was the shortest abundant fatty acid incorporated, indicating that DepT R -5 fabD mutant growth was not dependent on ai 15:0 or other short-chain fatty acids. Thus, the S. aureus fabD mutant can use diverse fatty acids, including those available in the host, and can dispense with branched chain fatty acids. These results indicate that the composition of the S. aureus membranes can be more flexible than generally supposed [24] , [27] , [32] , [43] . Role of the S. aureus fabD allele in FASII bypass To confirm that the fabD mutation is responsible for fatty acid dependency of DepT R -5, the wild type fabD gene was cloned in expression vector pJ (resulting in pJ-fabD) and established in the mutant strain background. To simulate in vivo conditions and obtain insight into S. aureus fabD mutant behaviour in the animal host, tests were performed in medium supplemented with liver and kidney extracts as fatty acid sources. In non-supplemented medium, the pJ-fabD plasmid restored ai 15:0 synthesis and growth to the DepT R -5 strain, confirming that the fabD mutation was responsible for the FASII defect ( Fig. 4a ). Importantly, growth of DepT R -5 (pJ) in host organ extracts was comparable to that of the Newman (pJ) strain, indicating that DepT R -5 can grow robustly while using exclusively host fatty acids. In this condition, complementation with pJ-fabD also resulted in ai 15:0 synthesis ( Fig. 4b ). In triclosan plus host organ extracts, growth of DepT R -5 (pJ-fabD) lagged slightly behind that of DepT R -5 (pJ) ( Fig. 4c , Supplementary Fig. 5a ). The intermediate effect could indicate that triclosan exerts a counter-selective effect on the plasmid-carried fabD copy. 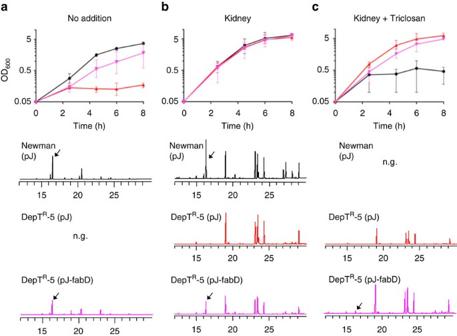Figure 4: Complementation of DepTR-5 by the wild typefabDallele. Overnight LB-FA cultures of WT and DepTR-5 strains carrying pJ (control plasmid), or pJ-fabD (expressing thefabDgene) were washed twice in LB, and cultures were inoculated at a starting OD600=0.05 in (a) LB (Cm 3 μg ml−1and ATc 50 ng ml−1), (b) the same medium containing sterile-filtered pig kidney extract (3% final volume) without or (c) with triclosan (0.5 μg ml−1). OD600was followed over 8 h. Fatty acid profiles were determined from harvested cells, as shown below the corresponding growth condition. N.g., no growth. Reference fatty acid profile and peak identification of kidney extract is inSupplementary Fig. 4. Growth results show the average with standard deviation of three experiments that gave comparable results (Supplementary Fig. 5). However, despite precautions, growth was variable between independent experiments, which may be due to the counter-selective effect of triclosan on the pJ-fabD plasmid. Figure 4: Complementation of DepT R -5 by the wild type fabD allele. Overnight LB-FA cultures of WT and DepT R -5 strains carrying pJ (control plasmid), or pJ-fabD (expressing the fabD gene) were washed twice in LB, and cultures were inoculated at a starting OD 600 =0.05 in ( a ) LB (Cm 3 μg ml −1 and ATc 50 ng ml −1 ), ( b ) the same medium containing sterile-filtered pig kidney extract (3% final volume) without or ( c ) with triclosan (0.5 μg ml −1 ). OD 600 was followed over 8 h. Fatty acid profiles were determined from harvested cells, as shown below the corresponding growth condition. N.g., no growth. Reference fatty acid profile and peak identification of kidney extract is in Supplementary Fig. 4 . Growth results show the average with standard deviation of three experiments that gave comparable results ( Supplementary Fig. 5 ). However, despite precautions, growth was variable between independent experiments, which may be due to the counter-selective effect of triclosan on the pJ-fabD plasmid. Full size image CondT R -17 grew both without and with fatty acid supplementation, and as expected, strong phenotypic differences were not observed in CondT R -17 complementation tests. The CondT R -17 (pJ or pJ-fabD) strains grew like Newman (pJ) in host organ extracts (data not shown). However, as above, CondT R -17 (pJ-fabD) displayed a slight growth retardation compared with CondT R -17 (pJ) in fatty-acid-triclosan-containing media as shown in the presence of kidney extracts ( Supplementary Fig. 5b ). In view of the absence of other mutations in the CondT R -17 strain, the identification of other ‘CondT R ’ isolates mutated in fabD ( Table 1 ), and the existence of fabD variants with FA-T R phenotypes among clinical isolates (below), we consider that fabD G196R is responsible for the CondT R -17 conditional phenotype. These results lead us to conclude that the fabD allele is responsible for the FASII defect in DepT R -5 and CondT R -17 strains. Both mutants grew comparably to the WT strain in host-simulated conditions, suggesting that these mutants would behave like the wild type strain in host compartments. Cross-resistance of S. aureus fabD mutants to FASII inhibitors AFN-1252 is a FabI inhibitor in clinical trials [44] ; platensimycin is a FabF inhibitor and antimicrobial candidate [11] . Cross-resistance between triclosan and these drugs was tested. S. aureus Newman (WT) and fabD mutants DepT R -5 and CondT R -17 were plated on BHI or BHI-FA media. FabI inhibitors triclosan and AFN-1252, and the FabF inhibitor platensimycin were spotted on lawns (at 100, 100 and 16 times the respective minimal inhibitory concentrations (MIC)) ( Fig. 5a–d ). Triclosan- and AFN-1252- resistant colonies appeared within the inhibitory zones of the WT strain only on fatty-acid-containing plates (compare Fig. 5a,b ). Platensimycin was poorly effective in both media at the tested concentration. We also noted a pronounced decrease in the inhibitory zone diameter for triclosan on BHI-FA compared with BHI plates (compare Fig. 5a,b ). In contrast, both DepT R -5 and CondT R -17 strains grew, albeit more slowly, within inhibitory zones of the 3 FASII inhibitors on BHI-FA plates ( Fig. 5c,d ). 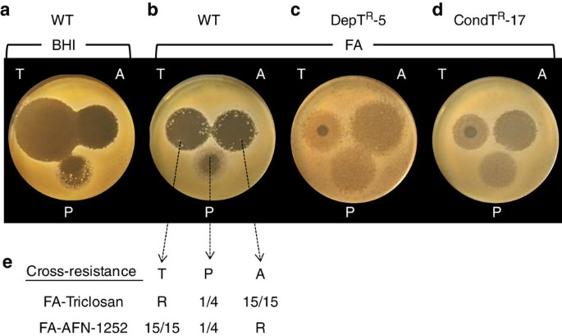Figure 5:S. aureuscross-resistance to anti-FASII drugs in the presence of exogenous fatty acids. Overnight BHI-FA-grown cultures of Newman WT, DepTR-5, and CondTR-17 were washed twice in BHI and plated on BHI solid medium without (a) (for Newman strain) or with fatty acids (b–d). Plates were spotted with triclosan (‘T’, 1.5 μg), AFN-1252 (‘A’, 1 μg), and platensimycin (‘P’, 8 μg), respectively 100, 100 and 16 times the MIC. Photographs were taken after 48 h at 37 °C. (c) DepTR-5 and (d) CondTR-17 strains accrue resistance to all three drugs on FA plates as seen by growth within the halo region, as compared with (b) the WT strain. The small inhibitory zone around triclosan is attributed to non-specific membrane effects12. (e) colonies that appeared within the inhibitory zones of WT strains on BHI-FA plates were cross-patched on BHI, BHI-FA, BHI-FA-AFN-1252 (80 ng ml−1) and FA-triclosan (250 ng ml−1). All colonies picked in fatty acids as triclosan-resistant were AFN-1252-resistant, and conversely. Fatty acid profiles (not shown) determined for colonies from each anti-FASII selective plate were fully exogenous. Figure 5: S. aureus cross-resistance to anti-FASII drugs in the presence of exogenous fatty acids. Overnight BHI-FA-grown cultures of Newman WT, DepT R -5, and CondT R -17 were washed twice in BHI and plated on BHI solid medium without ( a ) (for Newman strain) or with fatty acids ( b – d ). Plates were spotted with triclosan (‘T’, 1.5 μg), AFN-1252 (‘A’, 1 μg), and platensimycin (‘P’, 8 μg), respectively 100, 100 and 16 times the MIC. Photographs were taken after 48 h at 37 °C. ( c ) DepT R -5 and ( d ) CondT R -17 strains accrue resistance to all three drugs on FA plates as seen by growth within the halo region, as compared with ( b ) the WT strain. The small inhibitory zone around triclosan is attributed to non-specific membrane effects [12] . ( e ) colonies that appeared within the inhibitory zones of WT strains on BHI-FA plates were cross-patched on BHI, BHI-FA, BHI-FA-AFN-1252 (80 ng ml −1 ) and FA-triclosan (250 ng ml −1 ). All colonies picked in fatty acids as triclosan-resistant were AFN-1252-resistant, and conversely. Fatty acid profiles (not shown) determined for colonies from each anti-FASII selective plate were fully exogenous. Full size image Cross-resistance was then checked for colonies isolated from WT BHI-FA plates as triclosan, AFN-1252 or platensimycin resistant ( Fig. 5b ). Colonies were patched on BHI-FA medium containing triclosan (0.25 μg ml −1 ) or AFN-1252 (0.08 μg ml −1 ) ( Fig. 5e ). Fatty acid profiles of colonies as determined on primary selections and cross-selections were all exogenous (not shown). In addition, liquid cultures of DepT R -5 and CondT R -17 confirmed the capacity of DepT R -5 and CondT R -17 to grow on platensimycin and incorporate exogenous fatty acids ( Supplementary Fig. 6 ). These results further support a role of fatty acids in facilitating S. aureus escape from anti-FASII inhibition, and show that mutants selected by the use of a FASII inhibitor can be resistant to other FASII inhibitors. Infection by S. aureus fabD mutants Infections by fabD DepT R -5, fabD CondT R -17 or the WT strain were compared in a mouse sepsis model. A low inoculum (10 6 CFU) was used to avoid the possibility of false-positive virulence assignments [32] . The conditional FA-T R mutant, CondT R -17, was as infective as the parental Newman strain and gave equivalent CFUs in both liver and kidneys ( Fig. 6 ). These results indicate that this strain, and possibly similar variants, can retain full virulence. 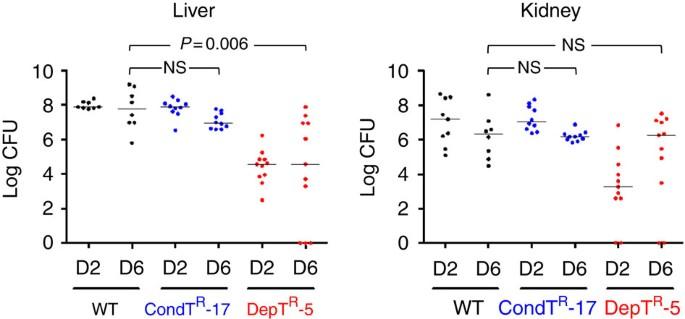Figure 6: Infection and persistence offabDisolates in a mouse model. Newman WT (black), CondTR-17 (fabDconditional; blue), and DepTR-5 (fabDfatty-acid-dependent; red) strains were prepared. 106CFU were injected in the tail veins of 6-week female BALB/c mice (in groups of 8–11). In these experiments, one WT-infected and one CondTR-17-infected mouse died 4 days post-infection. At days 2 (D2) and 6 (D6), animals from each group were sacrificed and dissected. Liver and kidney were homogenized by ultra-turrax and CFU per organ were determined by serial dilutions on BHI-FA plates containing 10% serum. Results are pooled from two independent experiments. Statistical tests were done using Mann–Whitney U to determine differences in CFU between groups on D2 and/or D6. No significant differences were observed between WT and CondTR-17 in any test condition. Notably, no significant difference was observed between WT and DepTR-5 CFUs in kidneys at D6 (P=0.77). NS, non-significant differences. The detection limit was 102CFU per organ; samples with no CFUs were plotted as ‘0’. In DepTR-5 samples, one mouse showed no detectable counts in liver or kidney. Figure 6: Infection and persistence of fabD isolates in a mouse model. Newman WT (black), CondT R -17 ( fabD conditional; blue), and DepT R -5 ( fabD fatty-acid-dependent; red) strains were prepared. 10 6 CFU were injected in the tail veins of 6-week female BALB/c mice (in groups of 8–11). In these experiments, one WT-infected and one CondT R -17-infected mouse died 4 days post-infection. At days 2 (D2) and 6 (D6), animals from each group were sacrificed and dissected. Liver and kidney were homogenized by ultra-turrax and CFU per organ were determined by serial dilutions on BHI-FA plates containing 10% serum. Results are pooled from two independent experiments. Statistical tests were done using Mann–Whitney U to determine differences in CFU between groups on D2 and/or D6. No significant differences were observed between WT and CondT R -17 in any test condition. Notably, no significant difference was observed between WT and DepT R -5 CFUs in kidneys at D6 ( P =0.77). NS, non-significant differences. The detection limit was 10 2 CFU per organ; samples with no CFUs were plotted as ‘0’. In DepT R -5 samples, one mouse showed no detectable counts in liver or kidney. Full size image The DepT R -5 mutant showed delayed kinetics of infection. At two days post-infection, significantly lower CFUs were present in both liver and kidneys compared with the WT strain ( P =0.001 in both organs using the Mann–Whitney U -test). However, these differences narrowed at 6 days post-infection, particularly in kidneys, where DepT R -5 CFUs increased and were not statistically different from WT CFUs ( P =0.77 in kidneys) ( Fig. 6 ). Colonies issued from the 6-day infection were confirmed to maintain fatty acid growth dependency, and two colonies selected at random from each organ were confirmed to carry the original fabD mutation. Our results indicate that both CondT R and DepT R mutants would resist challenge by a FASII inhibitor in vivo . As DepT R -5 and CondT R -17 also proliferate and incorporate fatty acids in the presence of AFN-1252 and platensimycin ( Fig. 5c,d ), we speculate that both types of mutants might override FASII inhibition regardless of the FASII inhibitor. FASII bypass in natural isolates carrying FabD polymorphisms Our results show that the CondT R -17 G196R substitution correlates with FASII bypass via incorporation of exogenous fatty acids. We searched public databases for natural S. aureus isolates carrying FabD modifications at the G196 position, and found three such isolates. Two independent sputum and nare isolates carry FabD R196 : M0251 (a methicillin-resistant S. aureus (MRSA) clonal complex CC5 isolate, BioSample accession code SAMN02325289) and M1532 (BioSample accession code SAMN02364048). The third strain, SA40, is a community- and epidemic-associated methicillin-resistant sequence type ST59 that was isolated from a healthy child and carries a FabD S196 protein. A closely related ST59 strain SA957 is an MRSA blood isolate that does not carry the FabD 196 polymorphism [45] . These S. aureus isolates as well as two FAT R mutants were tested for their capacity to bypass FASII. The three strains carrying FabD 196 polymorphisms, but not the Newman or SA957 strains, showed FASII bypass on BHI-FA-T liquid medium, as verified by growth and exogenous FA incorporation ( Table 2 ). These results further support the correlation between fabD 196 polymorphism and anti-FASII resistance, and show the capacity of S. aureus human isolates to use exogenous fatty acids to overcome FASII inhibitors. They also indicate that anti-FASII-resistance is present in some commensal and clinical isolates. Table 2 Natural clinical isolates bear fabD variants that favour FASII bypass. Full size table Redistribution of acyl-ACP pools in fabD variants FabD catalyses the transfer of malonyl from malonyl-CoA to acyl-carrier proteins (ACPs), yielding malonyl-ACP ( Supplementary Fig. 1 ). We considered that FabD polymorphisms near the active site (that is, position 196) might lower the efficiency of this reaction, thus leaving free ACP available for exogenous fatty acid incorporation. Two strain pairs were used to test this hypothesis: Newman strain ( fabD G196 )–CondT R -17 ( fabD R196 ) and ST59 clinical strains SA957 ( fabD G196 )–SA40 ( fabD S196 ). Cell extracts and culture supernatants were prepared from 4 h cultures in BHI-FA-T. Short- and long-chain acyl-ACP were assessed on Western blots of conformation-sensitive gels using anti-ACP antibodies [27] , [46] ; fatty acid profiles of cell extracts were done in parallel ( Fig. 7 ). A dithiothreitol (DTT)-treated extract of BHI-grown Newman strain was used to identify the migration position of free ACP [27] , [46] , [47] . 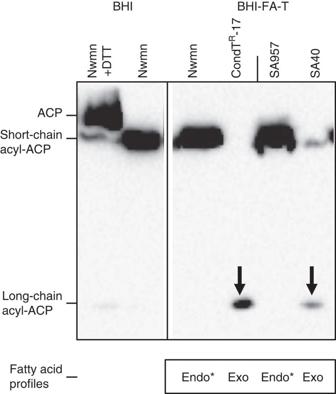Figure 7: Shift in ACP species in strains withfabD196polymorphisms. The impact of an altered amino acid at FabD position 196 on acyl-ACP pools was tested by comparing strain pairs: Newman and CondTR-17 (G196 and R196 respectively), and the ST59 pair SA957 (virulent) and SA40 (nasal isolate)45(G196 and S196 respectively). Extracts prepared from 4 h cultures in BHI-FA-T medium were run on conformation-sensitive gels. Anti-ACP antibodies were used to identify ACP moieties after gel transfer. In these gels, migration of acyl-ACP species increases with longer acyl chain length46,66. DTT treatment reduces acyl-ACP thioesters and releases free ACP47; the DTT-treated Newman protein extract from BHI-grown cells was used as migration control. Short-chain acyl-ACP is predominant in reference strains, and long-chain acyl-ACP moieties (arrows) are detected only in extracts offabDvariants. Results of fatty acid profiles of reference strains andfabDvariants are indicated below respective lanes. Nwmn, Newman strain; *, fatty acid profiles derived from non-growing cultures. The Western is from a single gel with the same exposure, and results are representative of 3 biologically independent experiments. The Western blot shown above corresponds to the entire gel. Figure 7: Shift in ACP species in strains with fabD 196 polymorphisms. The impact of an altered amino acid at FabD position 196 on acyl-ACP pools was tested by comparing strain pairs: Newman and CondT R -17 (G196 and R196 respectively), and the ST59 pair SA957 (virulent) and SA40 (nasal isolate) [45] (G196 and S196 respectively). Extracts prepared from 4 h cultures in BHI-FA-T medium were run on conformation-sensitive gels. Anti-ACP antibodies were used to identify ACP moieties after gel transfer. In these gels, migration of acyl-ACP species increases with longer acyl chain length [46] , [66] . DTT treatment reduces acyl-ACP thioesters and releases free ACP [47] ; the DTT-treated Newman protein extract from BHI-grown cells was used as migration control. Short-chain acyl-ACP is predominant in reference strains, and long-chain acyl-ACP moieties (arrows) are detected only in extracts of fabD variants. Results of fatty acid profiles of reference strains and fabD variants are indicated below respective lanes. Nwmn, Newman strain; *, fatty acid profiles derived from non-growing cultures. The Western is from a single gel with the same exposure, and results are representative of 3 biologically independent experiments. The Western blot shown above corresponds to the entire gel. Full size image Acyl-ACP species were redistributed in both fabD variants (CondT R -17 and SA40) compared with respective reference strains. Short-chain acyl-ACP pools were decreased in both variant strains, which is consistent with a reduced FabD activity as hypothesized. In addition, the fabD mutants contain long-chain acyl-ACPs that are not detected in reference strains, and their fatty acid profiles (but not those of the reference strains) are fully exogenous. Certain fatty acids are known to induce ACP release from S. aureus cells [38] ; however, we found that at 4 h, supernatants of all strains produced weak signals that did not differ significantly between strain pairs ( Supplementary Fig. 7 ). Thus, we hypothesize that the FabD R196 and FabD S196 mutant enzymes may be less active than FabD G196 , allowing free ACPs to be loaded with exogenous long-chain fatty acids that can then be incorporated into membrane phospholipids. The present work shows that a fatty-acid-rich environment can favour the emergence of S. aureus strains displaying resistance to multiple FASII inhibitors. Point mutations in fabD appear to facilitate FASII bypass by enhancing incorporation of exogenous fatty acids. Conditional (CondT R ) fabD mutants can grow normally, and can also bypass FASII in the presence of exogenous fatty acids, which suggests that they might be able to spread successfully in environments such as host organs. The S. aureus fabD mutants can use various fatty acid combinations ( Fig. 3 ). This flexibility indicates that, contrary to previous assumptions [24] , [27] , [43] , the branched-chain fatty acid requirement in S. aureus is not strict, as shown here for fabD 196 variants in laboratory and clinical strains from major lineages (CC8, CC5 and ST59). It may also help survival of anti-FASII-resistant bacteria in different host compartments that vary in fatty acid composition. Therefore, we propose that all these factors need to be considered when developing anti-FASII drugs for treating S. aureus infection [4] , [5] , [8] , [10] , [11] , [48] , [49] . In FASII-bypass conditions, fabD 196 variant strains show decreased levels of short-chain acyl-ACPs and increased levels of long-chain acyl-ACPs, in comparison with reference strains ( Fig. 7 ). The decrease in short-chain acyl-ACP is consistent with our proposal that FabD 196 variants may have reduced enzyme activity. We speculate that the detected long-chain acyl-ACP species correspond to exogenous fatty-acyl-ACP intermediates in phospholipid synthesis, which is consistent with the exogenous fatty acid profiles of fabD 196 variants ( Fig. 7 ). FASII bypass might depend on the outcome of competition for ACP between two enzymes at opposing ends of the pathway: the FASII initiation enzyme FabD (which uses ACP to synthesize malonyl-ACP) and the post-FASII termination enzyme PlsX (which catalyses the reversible formation of acyl-phosphate from acyl-ACP) [43] , [50] . Lower FabD activity would leave more ACP available for PlsX, to drive the reaction towards the synthesis of long-chain acyl-ACP (the phospholipid synthesis precursor) from exogenous fatty acids, and thus lead to FASII bypass ( Fig. 8 ). At present, this or other roles for long-chain acyl-ACP, for example, in modulating FASII enzyme activities, need to be demonstrated. 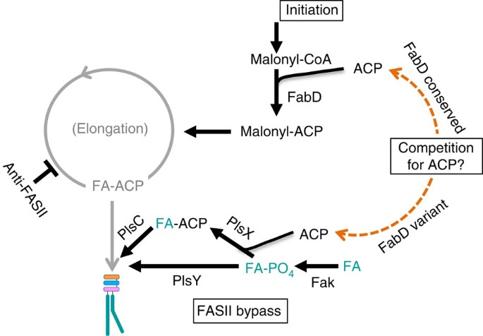Figure 8: Model of FASII bypass byS. aureus fabD196variants based on competition for ACP. A role for FabD in ACP balance and as a determining factor of FASII bypass is proposed. Indicated pathways and regulatory functions are as previously identified43,67. In grey, the inhibited FASII elongation pathway. FASII initiation enzyme FabD uses ACP and malonyl-CoA to synthesize malonyl-ACP50. In FASII inhibitory conditions, PlsX would compete for ACP pools to convert exogenous fatty acids (turquoise) into phospholipids. Less efficient activity of FabD196variants (Fig. 7) would leave ACP available for the PlsX reaction in the indicated direction (PlsX is a potentially reversible enzyme43), as indicated by orange dashed arrow. Fak-PlsY and Fak-PlsX-PlsC as proposed here, mediate acyl group joining respectively to positions 1 and 2 of the glycerol-3-phosphate (G3P) backbone31,43. FA, fatty acid; FA-ACP, acyl-ACP; FA-PO4, acyl-phosphate. Figure 8: Model of FASII bypass by S. aureus fabD 196 variants based on competition for ACP. A role for FabD in ACP balance and as a determining factor of FASII bypass is proposed. Indicated pathways and regulatory functions are as previously identified [43] , [67] . In grey, the inhibited FASII elongation pathway. FASII initiation enzyme FabD uses ACP and malonyl-CoA to synthesize malonyl-ACP [50] . In FASII inhibitory conditions, PlsX would compete for ACP pools to convert exogenous fatty acids (turquoise) into phospholipids. Less efficient activity of FabD 196 variants ( Fig. 7 ) would leave ACP available for the PlsX reaction in the indicated direction (PlsX is a potentially reversible enzyme [43] ), as indicated by orange dashed arrow. Fak-PlsY and Fak-PlsX-PlsC as proposed here, mediate acyl group joining respectively to positions 1 and 2 of the glycerol-3-phosphate (G3P) backbone [31] , [43] . FA, fatty acid; FA-ACP, acyl-ACP; FA-PO 4 , acyl-phosphate. Full size image Previous results showing that fatty acid auxotrophs carrying mutations in acc genes are avirulent led to the hypothesis that FASII-bypass mutants would not survive in the host [27] , [32] . In contrast, we have shown here that the fabD mutants DepT R -5 and CondT R -17 are infectious and persist in the host, and that clinical isolates chosen as bearing FabD 196 polymorphisms can bypass FASII inhibition ( Fig. 6 and Table 2 ). We speculate that this apparent discrepancy may be due to the different effects of the acc and fabD mutations on malonyl-ACP pools. FapR is a transcriptional repressor of FASII genes and of phospholipid synthesis genes plsX and plsC [51] ( Supplementary Fig. 1 ). FapR activity is alleviated by malonyl-CoA [51] , [52] , [53] . Mutations in acc leading to reduced synthesis of malonyl-CoA would result in FapR-mediated repression of phospholipid synthesis. On the contrary, malonyl-CoA would not be affected in the fabD mutants; it is even possible that the fabD mutants may accumulate malonyl-CoA, thus alleviating FapR-mediated repression of phospholipid synthesis genes. This situation would favour FASII bypass in environments rich in fatty acids. The present study uncovered fabD mutants as conferring a potentially non-deleterious anti-FASII escape strategy. It is possible that fabD mutations were not identified previously because of differences in experimental conditions, for example, in the choice of fatty acids and/or FASII inhibitors used in selections. Alternatively, strains might differ in their capacity to mediate FASII-bypass via mutations. Nevertheless, identification of fabD variant strains belonging to CC5, CC8, and ST59 groups and including MRSA isolates suggests that FASII-bypass variants may emerge in these dominant lineages. Our study revealed that FASII bypass mutants need not be fatty-acid auxotrophs. The CondT R mutant is resistant to several FASII inhibitors, yet grows normally and is infectious, indicating a gain of function. CondT R -like variants may thus present a risk of dissemination in the environment. The three tested clinical and commensal isolates with fabD 196 polymorphisms were all anti-FASII resistant ( Table 2 ). Among them, differential anti-FASII resistance of closely related ST59 strains SA40 (resistant) and SA957 (sensitive) that differ in fabD 196 further supports a role for fabD in FASII bypass among natural isolates. As FabD ORFs in genome-sequenced isolates are highly conserved within clonal types, we speculate that polymorphisms associated with FASII bypass arose by in vivo selection, possibly due to intensive use of triclosan in hygiene and household products [12] . A recent study of nasal secretions correlated the presence of triclosan with a greater incidence of colonizing S. aureus and consequent infection risk [18] . Interestingly, nasal secretions are fatty-acid-rich [54] , and the presence of triclosan or other FASII inhibitors could select for high frequency FASII bypass. The CondT R -like human nasal MRSA isolate (SA40) may be a case in point. DepT R -like mutants are also likely to be relevant to infection. Results presented here indicate that DepT R -5 persists in the kidney over a six-day infection period ( Fig. 6 ), indicating that these bacteria survive in the infected host. A recent study identified a FASII defect among clinical S. aureus small colony variants (SCV). SCV growth was restored to normal by fatty acid supplementation [55] , strongly pointing to a DepT R -like phenotype and implicating FASII bypass in chronic infection. Similar findings were reported for the opportunist pathogen Enterococcus faecalis [56] . Abscess formation during S. aureus infection is common, and it is tempting to speculate that this stage of infection may give privileged access to host fatty acids that support growth of both CondT R and DepT R mutants. Fatty-acid-rich skin [36] , [57] , possibly enriched by fatty-acid-containing skin products [58] , may be an ideal medium on which FASII inhibitors would select for FASII-bypass-competent staphylococci. The selection strategy used in our study mimicked this situation. Emergence of versatile S. aureus FASII bypass variants upon anti-FASII treatment may generate a long-term risk for persistence and infection [59] , requiring new rounds of antimicrobial therapy. Bacterial strains and growth conditions Experiments were performed using the S. aureus Newman strain [60] . SA40 (an Asian-Pacific nasal ST59 MRSA isolate from a healthy child) and SA957 (a virulent Taiwan ST59 blood isolate) were kindly provided by Freidrich Götz and Regine Stemmler (U. Tübingen, Germany) [45] . The M0251 (MRSA, clonal complex CC5) and M1532 strains are respectively nasal and sputum isolates that were generously provided by Mary Delaney and Michael Calderwood, and are part of the Brigham and Women’s Hospital collection (Boston, USA). Plasmid cloning and extraction were performed in E. coli strains Top10 (Invitrogen, France) and MG1655 (ref. 61 ). BHI and LB media were used for S. aureus , and LB for E. coli growth. The fatty-acid mixture (referred to as ‘FA’) comprises C14:0 (myristic acid), C16:0 (palmitic acid), and C18:1 (oleic acid); 100 mM stocks in dimethylsulphoxide (DMSO) of each fatty acid were mixed at a 1:1:1 ratio, and then diluted 1:200 for use in liquid or solid medium. Other fatty acid mixtures were prepared similarly, such that the final molar concentration of fatty acids was 0.5 mM (that is, 0.17 mM each fatty acid). All fatty acids were from Larodan Fine Chemicals (Sweden). Newborn calf serum (Sigma-Aldrich, France) and delipidated calf serum (Eurobio, France) were added to growth medium (10% final concentration) as indicated. Triclosan (Irgasan; Sigma-Aldrich) was routinely used at 0.25 μg per mL in liquid cultures; this is 15 times the MIC for S. aureus Newman strain in BHI medium. Platensimycin (Tebu-Bio, France) and AFN-1252 (MedChem Express) were used respectively at 2 μg ml −1 and 80 ng ml −1 as per published efficacies [11] , [27] . Anti-FASII drugs were prepared in DMSO. Kidney and liver extracts from adult pigs (usually 6 months, purchased at a local butcher shop) were prepared as follows: 200 g of each organ were cut in 0.5 cm cubes, and resuspended in PBS (1:2 w-v). Samples were homogenized using an ultra-turrax and then centrifuged twice (4,000 g for 30 min) to remove solid material. Supernatants were filtered through Whatman paper, recentrifuged at 20,000 g, and then sterile-filtered sequentially on 0.45 and 0.2 micron membranes. All steps were performed at 4 °C, and extracts were stored at −20 °C. Selection for triclosan resistance on FA plates Dilutions of overnight S. aureus Newman cultures were plated on four types of medium: non-selective (BHI); BHI plus FA (BHI-FA; FA are as described above); BHI with triclosan (BHI-T (0.25 μg ml −1 )), BHI containing FA and triclosan (BHI-FA-T (0.25 μg ml −1 )). Plates were incubated at 37 °C and scored at 48 h. Colonies were selected for phenotypic confirmation and characterization. Colony forming units (CFU) on plates were compared with determine FA-T R frequencies. Colonies that appeared on BHI-FA-T plates were then patched on the four plates as above to distinguish mutational phenotypes. Proportions of DepT R and CondT R mutants varied in independent experiments, possibly suggesting that slight variations in conditions may impact mutant phenotypes. Changes in fatty acid profiles of some FA-T R isolates were observed upon FA-T selection, particularly after storage, suggesting that adaptation might occur during selection and/or storage. Care was therefore taken in analysing profiles directly from selective plates and before storage. Determination of fatty acid profiles Whole cell esterified fatty acid determinations were done essentially as described [62] . Briefly, 1–2 ml S. aureus cultures (OD 600 =≥1) were centrifuged, washed once in 0.9% NaCl containing 0.02% Triton X-100, then washed twice in 0.9% NaCl. Cell pellets were treated with 0.5 ml of 1 N sodium methoxide. Heptane (200 μl) was then added, together with methyl-10-undecenoate (Sigma-Aldrich) as internal standard, vortexed for 1 min, and centrifuged. Fatty acid methyl esters were recovered in the heptane phase. Analyses were performed in a split-splitless injection mode on an AutoSystem XL Gas Chromatograph (Perkin-Elmer) equipped with a ZB-Wax capillary column (30 m × 0.25 mm × 0.25 μm; Phenomenex, France). Data were recorded and analysed by TotalChrom Workstation (Perkin-Elmer). S. aureus fatty acid peaks were detected between 12 and 30 min of elution. DNA sequencing The fabI , accABCD and fabD genes of selected S. aureus Newman strain FA-T R clones were sequenced. Primer pairs used for DNA amplification were: for fabI : FabIfd 5′-GATACAGAAAGGACTAAATCAAA-3′ and FabIrev 5′-TTTCCATCAGTCCGATTATTATA-3′ (ref. 20 ); for accDA : AccDAfd 5′-AACTAATGTATTGAATTGATGTAAACG-3′ and AccDArev 5′-AACATTCAACAGTCAAACGA-3′; for accBC : two sets were used AccBC1fd 5′-ACGGGTAGATGAAAACAAAC-3′ and AccBC1rev 5′-TCTTTTTCATCACGAGCAA-3′, and AccBC2fd 5′-AGTTGTTCCTGGTAGTGACG-3′ and AccBC2rev 5′-CCAGTGATGCCTTCGACTTC-3′; for fabD : FabDfd 5′-GAAGGTACTGTAGTTAAAGCACACG-3′ and FabDrev 5′-GCTTTGATTTCTTCGACTACTGCTT-3′. Whole genome sequencing was done on DepT R isolates DepT R -5, DepT R -72 and DepT R -45, CondT R mutant CondT R -17, and our parental Newman strain. Libraries were prepared with genomic DNA using the Illumina MiSeq next generation sequencing system (IMGM, Germany). The 2 × 250 base pair reads were aligned and sequence variations were analysed using CLC Genomics Workbench 5.5.2 software (CLC Bio). SNPs were found when comparing our control Newman strain to that in the Newman reference sequence (GenBank Nucleotide accession code NC_009641). Only differences between our laboratory Newman strain and FA-T R mutants were considered in genome comparisons. Cloning of fabD and acpP The fabD gene (locus NWMN_1140) and the fabD G196R variant gene were PCR-amplified from chromosomal DNA prepared from the Newman strain using the forward primer fabD-tail-F (5′-ATAAGCCGGGGGATCCACTAATGAGTAAAACAGCAATTATTTTTCCGGG -3′) and reverse primer fabD-tail-R (5′-GCGCGCAATTAACCCTCACTAAAGGGTTAGTCATTTTCATTC CATCCTTTCACATC-3′). Amplified DNA was cloned by Gibson assembly [63] . The vector, pJIM2246-ptetR [64] , was amplified for fabD cloning using primers pJ-fabD-R (5′-CCCGGAAAAATAATTGCTGTTTTACTCATTAGTGGATCCCCCG GCTTAT-3′) and pJ-fabD-F (5′-GATGTGAAAGGATGGAATGAAAATGACTAACCCTTTAGTGAGGGTTAATTGC GCGC-3′). Ligations were initially transformed into E. coli Top10. After plasmid verification by DNA sequencing, plasmids with and without inserts were transformed by electroporation into S. aureus strain RN4220 (ref. 60 ), re-extracted and transformed into Newman WT and fabD mutants. Standard electroporation protocols were followed [65] , except that DepT R -5 competent cells were prepared in BHI medium containing 10% heat-inactivated newborn calf serum and FA. The acpP gene (locus NWMN_1142) was cloned in plasmid pMalC4X (New England Biolabs) as a fusion to mbp . Briefly, acpP was PCR-amplified using forward primer 5′-GCGAATTCGAAAATTTCGATAAAGTAAAAGATATC-3′ and reverse primer 5′-GGGAAGCTTTTATTTTTCAAGACTGTTAATAAATTTAAC-3′. The digested fragment was then ligated to EcoRI-HindIII-linearized pMalC4X, and cloned in E. coli TG1, giving plasmid pMalC4X-acpP. Complementation tests Overnight cultures of wild type and fabD mutant strains carrying plasmids pJ or pJ-fabD were used to inoculate cultures at a starting density of OD 600 =0.05, in the following media: (i) LB containing 3 μg ml −1 Cm and 50 ng ml −1 anhydrotetracycline (ATc), (ii) same as (i) plus 10% kidney extract and (iii) same as (ii) plus 0.5 μg ml −1 triclosan. Growth was monitored in three independent experiments. Growth lags of DepT R -5 (pJ-fabD) in condition (iii) compared with DepT R -5 (pJ), and of CondT R -17 (pJ-fabD) compared with CondT R -17 (pJ) were determined as a ratio in individual experiments, and plotted as the ratio of the OD 600 values at different time points ( Supplementary Fig. 5 ). WT and fabD mutant resistance to FASII inhibitors WT, DepT R -5 and CondT R -17 strains were grown overnight in BHI-FA, washed twice in BHI, and 100 μl of OD 600 =0.1 bacterial suspension were plated on solid BHI or BHI-FA medium to obtain a lawn. Triclosan (1.5 μg in 3 μl), AFN-1252 (1 μg in 3 μl), and platensimycin (8 μg in 4 μl) were spotted immediately after plating. Plates were incubated at 37 °C and photographed after 48 h. Colonies growing within the inhibition zone of the anti-FASII drugs were patched to BHI, or to BHI-FA media containing or not triclosan 0.25 μg ml −1 , or AFN-1252 0.08 μg ml −1 , and scored for growth after 48 h. Bacterial patches were harvested directly for fatty acid profile evaluation. Mouse infection model Overnight cultures of DepT R -5, CondT R -17 and WT strains were grown in BHI-FA containing 10% serum. The morning of infection they were diluted to obtain a starting OD 600 =0.02 (WT and CondT R -17) and 0.04 (DepT R -5). Cells were grown in the same medium to OD 600 =1, washed, and resuspended in 0.9% NaCl to obtain 2 × 10 6 cells per mL, as confirmed by plating on BHI-FA plus 10% serum solid medium. Six-week female BALB/c mice (Janvier Labs, France) were injected in the tail vein with 10 6 cells in 500 μl 0.9% NaCl (8–11 animals per group). Animals were sacrificed at day 2 and day 6 (4–6 animals per time point) and dissected. Liver and kidneys were suspended in phosphate-buffered saline and homogenized with an ultra-turrax. CFUs were determined per organ type on BHI-FA plates containing 10% serum. DepT R -5 and CondT R -17 clones (20 for each mutant per organ), issued from day 6 platings, were randomly selected to verify fatty-acid-dependent and conditional phenotypes; conservation of the mutated alleles was further confirmed in two clones from each organ by PCR-sequencing. The presented data are pooled from animal studies performed as two independent experiments. Statistical analyses The Mann–Whitney U -test was used to evaluate whether differences in CFUs in mice infected by Newman or mutant derivatives were statistically significant. Differences were compared for day 2 or day 6 between Newman and mutant derivatives. Analyses were performed with GraphPad Prism Software Version 6.00 (GraphPad Software, USA). Statistical significance was given as P values. Growth capacity of fabD clinical variants and mutants on FA-triclosan Pre-cultures of Newman, M0251, M1532, SA957, SA40, CondT R -4, and CondT R -17 strains were prepared in BHI medium, and used to inoculate BHI or BHI-FA-T medium at an initial OD 600 =0.01. Cell density was determined as OD 600 measurements after 16 h growth. FA profiles were determined for cultures that reached OD 600 values above 0.5, which was defined as the growth threshold. Experiments were repeated three times. ACP assessment by conformation-sensitive gels Anti- S. aureus- ACP antibodies were prepared using ACP purified from E. coli TG1 carrying pMalC4X-acpP. For this purpose, cultures were grown in LB ampicillin (100 μg ml −1 ), and ACP-MBP expression was induced by IPTG 0.5 mM for 2 h during mid-exponential growth. The ACP-MBP fusion was recovered on a maltose resin and eluted with 20 mM maltose. The fusion protein was digested with Xa protease as per manufacturer’s instructions (New England Biolabs). Purified ACP was recovered from polyacrylamide gel electrophoresis–SDS (PAGE–SDS) gels and used for rabbit antibody preparation (Covalabs). The antibody preparation was validated on purified ACP protein, and used at 1:15,000 dilution. Conformation-sensitive (non-denaturing) gels were done as described [27] , [46] . Precultures of test strains were grown to OD 600 =0.5 in BHI medium at 37 °C. They were then split in equal aliquots, and further grown for 4 h in BHI or BHI-FA-T. Cultures were harvested for preparation of protein extracts as described [27] from the equivalent of OD 600 =5. DTT-treated extracts from BHI-grown S. aureus Newman were used as reference for the position of holo-ACP [27] , [47] . Samples (equivalent to OD 600 =0.25 in 10 μl) were loaded on 13% polyacrylamide gels containing 1 M urea, which were run at 100 volts for 3 h, and then transferred to PVDF membranes (0.2 μm; BioRad) for Western blotting and exposure using an ECL kit (Perkin-Elmer) as per supplier’s instructions. Ethics statement Animal experiments were performed at the animal facilities of HUPC in strict accordance with European Union guidelines for handling of laboratory animals, approved by the Ethics Committee for Animal Experimentation at the University of Paris-Descartes (CEEA 34), registration number 14-077. Data availability Genome sequence data for DepT R -5, DepT R -72, DepT R -45, CondT R -17, and our parental Newman strain have been deposited in the European Nucleotide Archive and can be accessed at http://www.ebi.ac.uk/ena/data/view/PRJEB11476 . The authors declare that all other data supporting the findings of this study are available within the article and its Supplementary Information files, or from the corresponding author upon request. How to cite this article: Morvan, C. et al . Environmental fatty acids enable emergence of infectious Staphylococcus aureus resistant to FASII-targeted antimicrobials. Nat. Commun. 7, 12944 doi: 10.1038/ncomms12944 (2016).